Holographic detection of the orbital angular momentum of light with plasmonic photodiodes Metallic components such as plasmonic gratings and plasmonic lenses are routinely used to convert free-space beams into propagating surface plasmon polaritons and vice versa. This generation of couplers handles relatively simple light beams, such as plane waves or Gaussian beams. Here we present a powerful generalization of this strategy to more complex wavefronts, such as vortex beams that carry orbital angular momentum, also known as topological charge. This approach is based on the principle of holography: the coupler is designed as the interference pattern of the incident vortex beam and focused surface plasmon polaritons. We have integrated these holographic plasmonic interfaces into commercial silicon photodiodes, and demonstrated that such devices can selectively detect the orbital angular momentum of light. This holographic approach is very general and can be used to selectively couple free-space beams into any type of surface wave, such as focused surface plasmon polaritons and plasmonic Airy beams. Photodetectors are widely used optical components that record the intensity of incident light by converting it into an electrical signal. In the detection process, any information about the phase profile of the incident wavefront is lost. Here we present a new approach to designing detectors, based on the principle of holography, which enables the detection of the number of twists of the wavefront within a wavelength of propagation—known as the topological charge of corkscrew-shaped wavefronts, characteristic of beams carrying orbital angular momentum (OAM)—while simultaneously taking advantage of widely available photodiode technology. The principle of holography, developed first in 1947 by Gabor [1] , was applied to free-space optical beams with the advent of the laser and later extended to surface waves by Cowan [2] in 1972. Holography is originally an imaging technique that consists of scattering an incident laser beam from an optically recorded interference pattern (the hologram) such that the scattered light reconstructs the three-dimensional image of an object. In the work of Cowan [2] , holograms were generated using surface waves as reference beams. In subsequent papers, authors made use of the collective excitation of free-electrons on metal surfaces [3] , known as surface plasmon polaritons (SPPs) to create and record holograms [4] , [5] , [6] . The interference between the light scattered by the object and the reference SPP beam creates high-intensity lines that imprint a phase grating onto the photographic film placed in contact with the metal surface. The information encoded in the film is reconstructed by sending a readout SPP beam propagating at the interface between the metal and the photographic film. In this paper, we demonstrate the use of the holography principle to design couplers for complex wavefronts. In particular, our approach simplifies the problem of recording the hologram by patterning it directly onto the device, thus removing the photographic layer commonly used in holography [7] . The hologram consists of a distribution of scatterers disposed directly onto the metal surface in the locations where constructive interference between the two waves occurs, that is, where the phase of both the incident wave and the SPP are equal. As an example of this powerful method, we have created holographic surfaces by interfering a converging SPP wave with incoming free-space beams carrying OAM, also known as optical vortex beams. Following the principle of reciprocity, these surfaces can scatter a diverging SPP wave into a free-space optical vortex beam as well. Vortex beams have a doughnut-like transverse intensity profile and carry an OAM of ħL i per photon, where L i is the topological charge and ħ is the reduced Planck's constant. OAM states are orthogonal and beams with different OAM can propagate collinearly while carrying a quantum number of any integer value. These intriguing properties make light with OAM appealing for applications in microscopy, optical trapping and optical communication [8] , [9] , [10] , [11] . To fully exploit the potential of OAM, several techniques have been developed to selectively detect it. Inspired by the pioneering work of Beth [12] on the detection of spin angular momentum, He et al . [13] measured the torque induced by OAM transferred from a vortex beam to absorptive particles. A more direct solution consists of reversing the wavefront using appropriate holographic plates [14] . The efficiency of such diffracting devices has been improved by an alternative mode-sorting approach, which combines interferometry and conjugate helical phase elements by directing photons with OAM states onto a series of output ports [10] . More evolved holographic plates can also simultaneously detect a large number of OAM states using a CCD camera [15] . Refractive elements have been recently developed to transform the OAM information into transverse momentum information for efficient detection of OAM with high quantum numbers with sensitivity down to the single photon limit [16] . All of these free-space methods require bulky systems comprising multiple components, which are usually not cost effective and are difficult to implement. Integrated photonic waveguide plates have been recently proposed to sort the OAM on-chip by sampling the wavefront of vortex beams using vertical gratings that couple light into phased-array waveguides [17] . In this paper, we propose a straightforward but powerful alternative approach to selectively detecting the OAM of light with a specific topological charge L i , using state-of-the-art commercial detectors integrated with couplers. This novel integration scheme is based on holographic interfaces which couple incident light into focusing SPPs. Holographic designs of SPP couplers for beams with OAM The schematic in Fig. 1a explains the procedure followed for the design of the holograms. We compute the in-plane interference pattern which occurs when a propagating and focused SPP coherently interacts with a single charged free-space vortex beam impinging on the interface at normal incidence ( Fig. 1b ). 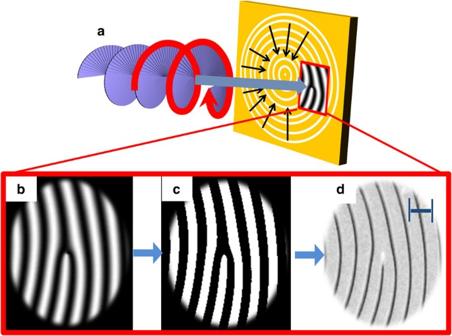Figure 1: Interferometric design of the plasmonic couplers. (a) Schematic explaining the approach used to design our holographic interfaces. Holographic couplers are designed by considering the interference between an incident beam with some complex wavefront, such as a vortex beam with a topological chargeLi=−1, impinging on the metal interface at normal incidence and a converging SPP beam. (b) Computer-generated interferogram. The incident vortex beam is assumed to be a Gaussian-vortex beam. (c) Binary version of the interferogram in panelb. The bright lines represent the locations of equal phase of the two beams, where maximum constructive interference occurs. (d) Scanning electron micrograph of a fabricated holographic interface where the grooves are placed at the equi-phase locations. Scale bar, 1 μm. The vortex beam is assumed to be Figure 1: Interferometric design of the plasmonic couplers. ( a ) Schematic explaining the approach used to design our holographic interfaces. Holographic couplers are designed by considering the interference between an incident beam with some complex wavefront, such as a vortex beam with a topological charge L i =−1, impinging on the metal interface at normal incidence and a converging SPP beam. ( b ) Computer-generated interferogram. The incident vortex beam is assumed to be a Gaussian-vortex beam. ( c ) Binary version of the interferogram in panel b . The bright lines represent the locations of equal phase of the two beams, where maximum constructive interference occurs. ( d ) Scanning electron micrograph of a fabricated holographic interface where the grooves are placed at the equi-phase locations. Scale bar, 1 μm. Full size image known as a Gaussian-vortex beam, characterized by a spiral wavefront of topological charge L i , where A ( r , z ) is the transverse Gaussian beam profile, r is the radial distance from the beam centre and z is the axial distance from the beam waist. In Fig. 1c , we compute the binary version of the hologram and in Fig. 1d , we show a micrograph of a holographic interface fabricated by focused ion beam (FIB) milling. Our structures were designed to work for visible light at a wavelength of 633 nm. Because of the transverse magnetic character of SPP modes, only the in-plane component of the SPP polarization can interfere with the incident light, which implies that about 10% of the SPP energy participates in the process. In Fig. 2 , we show two device designs: a coupler to convert an incident vortex beam of a given topological charge into a focused SPP wave and a conventional plasmonic lens for an incident Gaussian beam [18] , [19] , [20] . The performance of both structures is explored via finite-difference time-domain (FDTD) simulations using commercial software (Lumerical FDTD). Light coming at normal incidence is focused from the substrate side onto the apertured holographic interface. Then, it is coupled to a particular SPP mode and eventually propagates at the gold–air interface. In accordance with the design, the classical plasmonic lens efficiently focuses only the incident Gaussian beam, whereas the holographic fork-like coupler L g =1, designed for L i =−1, focuses only the incident light with this particular topological charge. 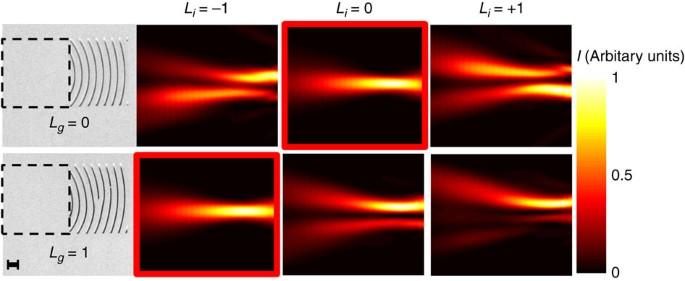Figure 2: Numerical simulations of the SPP intensity distribution. FDTD simulations of the intensity distribution of SPPs (in the plane of the metallic pattern), generated by illuminating the plasmonic holograms at normal incidence with a Gaussian beam and vortex beams of topological chargesLi=1 andLi=−1 with a Gaussian transverse intensity profile. The simulated field intensity distributions are displayed for the region immediately to the left of the gratings, identified with the dashed squares in the scanning electron microscopy image. In the first row, the hologram is created by interference of a converging SPP beam and a normally incident Gaussian beam, which can therefore launch a focused SPP beam when the Gaussian beam is normally incident on the hologram. When the incident wavefront is instead helical, characterized by a non-zero OAM, the hologram launches surface waves that do not interfere constructively along the symmetry axis of the device and therefore are not properly focused. Conversely in the second row, when the hologram is designed for an incident vortex beam of well-defined and non-zero OAM, the SPP beam is correctly focused by the structure when illuminated with the correct topological charge (Li=−1, second row).Lgis the angular momentum provided by the coupler to the incident beam as discussed in the text. In all of the simulations, light is incident from the substrate side (SiO2) atλ=633-nm at normal incidence. The period of the grooves is ~600-nm in accordance with the wavelength of SPPs but spatially varies according to the interference pattern; seeFig. 1b. Scale bar, 1-μm. Figure 2: Numerical simulations of the SPP intensity distribution. FDTD simulations of the intensity distribution of SPPs (in the plane of the metallic pattern), generated by illuminating the plasmonic holograms at normal incidence with a Gaussian beam and vortex beams of topological charges L i =1 and L i =−1 with a Gaussian transverse intensity profile. The simulated field intensity distributions are displayed for the region immediately to the left of the gratings, identified with the dashed squares in the scanning electron microscopy image. In the first row, the hologram is created by interference of a converging SPP beam and a normally incident Gaussian beam, which can therefore launch a focused SPP beam when the Gaussian beam is normally incident on the hologram. When the incident wavefront is instead helical, characterized by a non-zero OAM, the hologram launches surface waves that do not interfere constructively along the symmetry axis of the device and therefore are not properly focused. Conversely in the second row, when the hologram is designed for an incident vortex beam of well-defined and non-zero OAM, the SPP beam is correctly focused by the structure when illuminated with the correct topological charge ( L i =−1, second row). L g is the angular momentum provided by the coupler to the incident beam as discussed in the text. In all of the simulations, light is incident from the substrate side (SiO 2 ) at λ =633-nm at normal incidence. The period of the grooves is ~600-nm in accordance with the wavelength of SPPs but spatially varies according to the interference pattern; see Fig. 1b . Scale bar, 1-μm. Full size image Conservation of OAM and physical interpretation Because in the detection process incident light carrying OAM is converted into SPPs which carry no OAM, it is useful to consider how angular momentum is conserved in the course of the interaction with the structured metallic surface. This is conceptually a phase-matching process analogous to what occurs in a standard plasmonic coupler, made of periodic corrugations, which couples an incident plane wave to a SPP by providing a wavevector parallel to the surface, of magnitude inversely proportional to the grating period so that the tangential wavevector is conserved in the interaction. Recent experiments have shown that plasmonic metasurfaces consisting of suitably arranged metallic nanostructures can be designed to impart to the scattered wavefront an OAM of any topological charge [21] , [22] . In the present work, instead, we excite focused SPPs on the metallic nanostructured surfaces using optical vortex beams. One can understand this process in terms of conservation of angular momentum. Assuming a vortex beam (equation (1)), angular momentum conservation requires L i + L g =0, where L g is provided by the holographic coupler to cancel L i . Physically, the plasmonic lens with a fork-like dislocation fringe appearing at its centre is designed to impart an opposite OAM to the incident vortex beam so that it can excite a surface wave with no OAM, that is, a focused SPP. By design, the incident vortex beam ( L i =−1) converts into a SPP, which focuses along the axis of the device where an array of sub-wavelength holes funnels the light through the gold film towards the surface of the photodiode (schematic in Fig. 3a ). The sub-wavelength array of holes is placed in the focal region of the plasmonic coupler to act as a spatial filter. This coupler is positioned at the correct distance from the hologram to allow for preferential transmission through the holes of the focused SPP generated by a vortex beam of specific OAM. To avoid direct coupling of light into the detector, we choose the grating period to be much smaller than the SPP wavelength. The size of the holes is also sub-wavelength, to funnel light into the diode via extraordinary optical transmission [23] , [24] . An incident beam with the correct OAM will be focused at the centre of the device, whereas beams with any other topological charge will be defocused away from the array of holes and hence will not be detected. 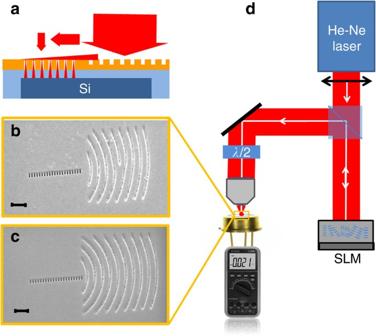Figure 3: Experiment to detect the OAM with patterned photodiodes. (a) Cross section of the patterned photodiodes. The holographic interface couples incident radiation into SPPs, which are then funneled as light into the detector by an array of sub-wavelength holes. The figure also shows the electron micrographs (scale bar, 1 μm) of two holograms patterned on top of the detectors: (b) (Lg=1) is designed to focus a vortex beam with OAMLi=−1 onto the array of holes and (c) (Lg=0) is a conventional plasmonic lens that focuses a Gaussian beam withLi=0. (d) The function of the spatial lightwave modulator (SLM) is to impart to the incident laser beam a spiral-shaped wavefront of well-defined OAM. A halfwave plate is used to control the incident polarization. The generated photocurrent is measured with a Keithley model 2400 ammeter. Figure 3b is an electron micrograph of the device with L g =−1, whereas Fig. 3c presents the one with L g =0. Figure 3: Experiment to detect the OAM with patterned photodiodes. ( a ) Cross section of the patterned photodiodes. The holographic interface couples incident radiation into SPPs, which are then funneled as light into the detector by an array of sub-wavelength holes. The figure also shows the electron micrographs (scale bar, 1 μm) of two holograms patterned on top of the detectors: ( b ) ( L g =1) is designed to focus a vortex beam with OAM L i =−1 onto the array of holes and ( c ) ( L g =0) is a conventional plasmonic lens that focuses a Gaussian beam with L i =0. ( d ) The function of the spatial lightwave modulator (SLM) is to impart to the incident laser beam a spiral-shaped wavefront of well-defined OAM. A halfwave plate is used to control the incident polarization. The generated photocurrent is measured with a Keithley model 2400 ammeter. Full size image Experimental results Figure 3d illustrates the experimental set-up used to characterize our integrated OAM detectors. The results of our experiment are summarized in Fig. 4 . 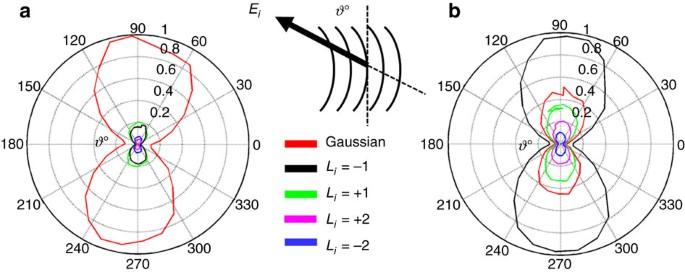Figure 4: Detected photocurrent as a function of the incident polarization and OAMs. Photocurrent is measured for two different holographic photodiodes, one patterned with a classical plasmonic lens (Fig. 3d,Lg=0) that focuses a Gaussian beam (a) and the other with a plasmonic lens (Fig. 3c,Lg=1) that focuses a vortex beam withLi=−1 (b). Each colour denotes a vortex beam incident with a different topological charge. The inset shows the orientation of the polarization of the incident electric field with respect to the grooves. Figure 4a shows the response of a photodiode patterned with a hologram created by the interference between a converging SPP and a Gaussian beam. Figure 4b presents the same measurements as in Fig. 4a but obtained using a photodiode patterned with the hologram designed by interference of converging SPP and an incident vortex beam of charge L i =−1. In Fig. 4a , the maximum photocurrent is observed for an incident Gaussian beam, that is, when the incident beam matches the design of the hologram, and the signal decreases considerably (below 10%) for beams with OAM. Conversely, Fig. 4b shows that the maximum photocurrent is measured for an incident vortex beam with L i =−1. Figure 4: Detected photocurrent as a function of the incident polarization and OAMs. Photocurrent is measured for two different holographic photodiodes, one patterned with a classical plasmonic lens ( Fig. 3d , L g =0) that focuses a Gaussian beam ( a ) and the other with a plasmonic lens ( Fig. 3c , L g =1) that focuses a vortex beam with L i =−1 ( b ). Each colour denotes a vortex beam incident with a different topological charge. The inset shows the orientation of the polarization of the incident electric field with respect to the grooves. Full size image We varied the incident polarization and we confirmed that, for both photodiodes, the maximum signal is obtained for an incident polarization oriented normal to the grooves of the holographic interface, that is, when the coupling to SPPs is maximized. The OAM conservation condition previously discussed implies that the centre of the vortex beam must be correctly aligned with the edge of the dislocation in the holographic coupler. We studied the effect of lateral displacements with respect to the centre of the hologram. The results of these simulations show that the OAM selectivity of the detector remains reasonable, even for lateral displacements ( Supplementary Fig. S1 ). In this work, we used standard silicon-based photodiodes which have a very large active area (about 13 mm 2 ) and exhibit a responsivity ~200 mA W −1 at λ =633 nm. Once patterned, the device performance is considerably degraded, with measured responsivity in the tens of microamps per watt. There are several reasons for this: first, we only detect light that is funneled through the sub-wavelength apertures. From FDTD simulations, we estimate that around 5% of the incident power coupled to the SPP is transmitted through the interface, eventually exciting SPPs on the other side of the interface and free-space photons. Only the free-space photons on the backside of the substrate are detected by the photodiode. We estimate from simulations that around 2% of the incident light reaches the detector ( Supplementary Fig. S2 ). It is important to point out that the wavelength used for the experiment is close to the intra-band absorption in gold where losses are considerable, thus shortening the SPPs propagation distance. This has several implications: it limits not only the size of the gratings but also the length of the array of holes to the SPP propagation length ( Supplementary Fig. S3 ); thus, only a small portion of the photodiode is actually used for the detection. Detection of OAM can be achieved with substantially higher efficiencies at longer wavelengths, especially for the frequencies in the region of interest for optical communications [25] . Note that by replacing the detector with an avalanche photodiode, one could increase the responsivity by a factor ~10 3 up to ~1 mA W −1 . Detection of higher OAM can be achieved with good selectivity by modifying the holographic coupler; see the example in Supplementary Fig. S4 with a doubly charged OAM detector. Further increase of the selectivity between adjacent OAMs would require precise tailoring of the transmitting array of holes as discussed in Supplementary Fig. S4 . In conclusion, we demonstrated a new technique for the design of plasmonic couplers for beams with OAM. The concept, inspired by the principle of holography, relies on coherent scattering of light from free space into SPPs by patterning suitable grooves at locations where the two beams have the same phase. We demonstrated that holographic surfaces can convert free-space laser beams with different topological charges into focused SPP waves. In this way, we extended the functionality of a standard photodiode, enabling the sorting of the various incident OAM states of light. The holographic method of generating plasmonic couplers has potential for applications in various areas of integrated optics and can be used, in a straightforward way, to design other interfaces, for example, for the generation of plasmonic non-diffracting beams [26] , [27] . Detector fabrication We patterned our vortex hologram on the front window of commercially available silicon detectors, which were first coated with a 200-nm-thick gold film using electron beam evaporation. The shallow grooves forming the hologram were defined by FIB milling (Zeiss NVision 40). The groove width is ~150-nm, 75-nm deep (halfway through the gold film) and the spacing is given by the simulated interference pattern, as discussed in the introduction. A second FIB milling is performed at higher exposure to create an array of sub-wavelength holes in the focal region of the plasmonic coupler. As the holes pierce all the way through the gold film, the holes spacing is chosen as ~200-nm, which is smaller than the free-space wavelength to avoid direct coupling of the light into the detector. OAM measurements A TEM 00 laser mode of a linearly polarized He-Ne laser, emitting at 633-nm, is incident on a programmable spatial lightwave modulator (Hamamatsu LCOS-SLM X 10468) to modify its OAM and is later directed to the silicon photodetector (Hamamatsu S2386-18K). A halfwave plate is inserted along the beam path to control the polarization of the incident light onto the detector. The current is monitored at the photodiode with a Keithley model 2400. How to cite this article: Genevet, P. et al . Holographic detection of the orbital angular momentum of light with plasmonic photodiodes. Nat. Commun. 3:1278 doi: 10.1038/ncomms2293 (2012).